PI 3-kinase-dependent phosphorylation of Plk1–Ser99 promotes association with 14-3-3γ and is required for metaphase–anaphase transition Polo-like kinase 1 (Plk1) controls multiple aspects of mitosis and is activated through its phosphorylation at Thr210. Here we identify Ser99 on Plk1 as a novel mitosis-specific phosphorylation site, which operates independently of Plk1–Thr210 phosphorylation. Plk1–Ser99 phosphorylation creates a docking site for 14-3-3γ, and this interaction stimulates the catalytic activity of Plk1. Knockdown of 14-3-3γ or replacement of wild-type (WT) Plk1 by a Ser99-phospho-blocking mutant leads to a prometaphase/metaphase-like arrest due to the activation of the spindle assembly checkpoint. Inhibition of phosphatidylinositol 3-kinase (PI3K) and Akt significantly reduces the level of Plk1–Ser99 phosphorylation and delays metaphase to anaphase transition. Plk1–Ser99 phosphorylation requires not only Akt activity but also protein(s) associated with Plk1 in a mitosis-specific manner. Therefore, mitotic Plk1 activity is regulated not only by Plk1–Thr210 phosphorylation, but also by Plk1 binding to 14-3-3γ following Plk1–Ser99 phosphorylation downstream of the PI3K–Akt signalling pathway. This novel Plk1 activation pathway controls proper progression from metaphase to anaphase. The genetic stability of all eukaryotes depends largely on error-free segregation of chromosomes in mitosis and perturbation of this process can lead to aneuploidy, a major cause of cancer [1] , [2] . Chromosome segregation is controlled by the activities of mitotic kinases, notably cyclin-dependent kinase 1 (Cdk1), and orthologues of Drosophila melanogaster Aurora (A–C types) and polo-like kinase 1 (Plk1) [3] , [4] , [5] , [6] . Among these mitotic kinases, Plk1 regulates multiple aspects of spindle assembly including bipolar spindle formation [7] , [8] , [9] . From prophase to metaphase, Plk1 is targeted to centrosomes and kinetochores (KTs). A major role of Plk1 at the centrosomes is to promote the increased nucleation of microtubules (MTs), a process known as centrosome maturation. At KTs, Plk1 is required for the establishment of stable KT–MT interactions. Thus, compromising Plk1 function in human cells leads to a prominent prometaphase/metaphase-like arrest, which is dependent on the activation of the spindle assembly checkpoint (SAC). Plk1 activation requires phosphorylation on Thr210 within the activation T-loop in the catalytic domain. During mitosis, two members of the Aurora kinase family are known to regulate Plk1–Thr210 phosphorylation and activation. At the centrosomes, Aurora A (AurA) phosphorylates Plk1 on Thr210 in a Bora-dependent manner and this controls entry into mitosis especially after DNA damage/replication-checkpoint-dependent arrest [10] , [11] . At the centromeres, the inner centromere protein (INCENP) acts as a platform for the cross-talk between Aurora B (AurB) and Plk1. Complex formation between these proteins is required not only for Plk1–Thr210 phosphorylation by AurB, but also for Plk1 function at the KT [12] . In this study, we show that Plk1 binds to 14-3-3γ specifically during mitosis. This binding stimulates Plk1 catalytic activity without affecting the phosphorylation status of Plk1–Thr210. These phenomena are controlled by Plk1 phosphorylation on a novel site, Ser99. Plk1–Ser99 phosphorylation largely depends on the activities of phosphatidylinositol 3-kinase (PI3K) and Akt (also called protein kinase B). The perturbation of this pathway activates the SAC, which significantly delays the time from metaphase to anaphase. Identification of 14-3-3γ as a novel regulator of mitosis We previously reported that 14-3-3γ participates in the DNA damage response through the modulation of a signalling pathway that links Chk1 to Cdc25A [13] , [14] . In order to examine whether 14-3-3 proteins are also involved in cell-cycle progression in the absence of exogenously introduced DNA damage, we examined the effects of 14-3-3 knockdown by transfection with short interfering RNAs (siRNAs) specific for each 14-3-3 subtype. For each protein, we targeted two independent sequences. Immunoblotting with antibodies against each subtype (characterized in Supplementary Fig. S1a ) indicated the successful depletion of each subtype of 14-3-3 ( Supplementary Fig. S1b ). As judged by morphological features and mitotic marker phosphorylation (histone H3-Ser28 phosphorylation) [15] , 14-3-3γ depletion increased the mitotic index, whereas the depletion of other subtypes had only marginal effects ( Fig. 1a ). To examine this phenomenon more precisely, we combined siRNA transfection with double-thymidine block (DTB) synchronization [16] . In cells treated with control siRNA (siControl), the mitotic index reached a peak at 11 h after release from a second thymidine block and rapidly decreased thereafter. However, the decline in mitotic index was severely impaired in cells treated with 14-3-3γ-specific siRNA (si14-3-3γ), whereas we observed only marginal changes in the timing of mitotic entry and the height of the mitotic index peak ( Fig. 1b ). Next, we performed live-cell imaging assays using HeLa cells stably expressing histone H2B-GFP (green fluorescent protein) [17] . Control cells proceeded rapidly from nuclear envelope breakdown to anaphase onset (mean of 36 min; Fig. 1c and Supplementary Movie 1 ), whereas 14-3-3γ depletion yielded a significant increase in this duration (target sequence #1, mean of 153 min; #2, mean of 113 min; Fig. 1c and Supplementary Movie 2 ). These results suggested that 14-3-3γ depletion leads to a prometaphase/metaphase-like arrest. 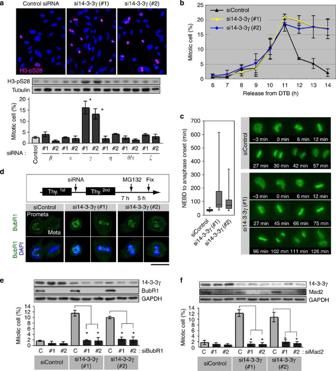Figure 1: 14-3-3 protein controls proper SAC inactivation in a γ-subtype-dependent manner. (a) Forty-eight hours after transfection with an indicated siRNA, HeLa cells were stained with anti-H3-pSer28 (red) and 4',6-diamidino-2-phenylindole (blue). Immunoblotting with anti-H3-pSer28 and anti-α-tubulin (loading control) are also shown in insets. (b) The effect of 14-3-3γ knockdown on cell-cycle progression after DTB synchronization. (c) Live-cell imaging analyses using H2B-GFP-expressing HeLa cells. Box-and-whisker plots show the elapsed time that cells spent in mitosis from nuclear envelope breakdown (t=0) to anaphase onset (n≥60 from two independent experiments). (d) The effect of 14-3-3γ silencing on KT-associated BubR1. Scale bar, 10 μm. (e, f) The effects of BubR1 or Mad2 silencing on mitotic arrest induced by 14-3-3γ depletion. Mitotic indices are shown as mean±s.e.m. from three independent experiments (n>200 each). *P<0.01; Student’st-test. Figure 1: 14-3-3 protein controls proper SAC inactivation in a γ-subtype-dependent manner. ( a ) Forty-eight hours after transfection with an indicated siRNA, HeLa cells were stained with anti-H3-pSer28 (red) and 4',6-diamidino-2-phenylindole (blue). Immunoblotting with anti-H3-pSer28 and anti-α-tubulin (loading control) are also shown in insets. ( b ) The effect of 14-3-3γ knockdown on cell-cycle progression after DTB synchronization. ( c ) Live-cell imaging analyses using H2B-GFP-expressing HeLa cells. Box-and-whisker plots show the elapsed time that cells spent in mitosis from nuclear envelope breakdown ( t =0) to anaphase onset ( n ≥60 from two independent experiments). ( d ) The effect of 14-3-3γ silencing on KT-associated BubR1. Scale bar, 10 μm. ( e, f ) The effects of BubR1 or Mad2 silencing on mitotic arrest induced by 14-3-3γ depletion. Mitotic indices are shown as mean±s.e.m. from three independent experiments ( n >200 each). * P <0.01; Student’s t -test. Full size image After DTB synchronization and siRNA treatment, we arrested the cells at metaphase by using the proteasome inhibitor MG132 and monitored the KT-association of BubR1, a marker of SAC activity [18] , [19] . In control cells, BubR1 was localized at KTs in prometaphase (before chromosome alignment), and then dissociated from KTs in metaphase (when all chromosomes were aligned at the metaphase plate). However, in the case of 14-3-3γ-depletion, strong BubR1 signals were observed on KTs in the majority of mitotic cells, even in cells where all chromosomes appeared to be aligned at the equatorial plane ( Fig. 1d ). In addition, the increase in mitotic index was reversed by the silencing of BubR1 ( Fig. 1e ) or Mad2 ( Fig. 1f ), which causes inactivation of the SAC [18] , [19] . These results indicate that the knockdown of 14-3-3γ prolongs mitosis in a SAC-dependent manner. 14-3-3γ activates Plk1 specifically in mitosis As 14-3-3 is known as a scaffold protein [20] , [21] , we searched for binding partners of 14-3-3γ in mitosis. By the combination of glutathione S- transferase (GST) pull-down and mass spectrometry/mass spectrometry analyses, we identified several putative proteins, which bound to GST-14-3-3γ in a mitosis-specific manner ( Fig. 2a ). Among these proteins, we focused on Plk1 because the phenotype of 14-3-3γ depletion ( Fig. 1 ) closely resembled that of Plk1 depletion and other identified proteins were already reported to interact with other subtypes of 14-3-3 [22] , [23] . Immunoblotting with anti-Plk1 confirmed that Plk1 was indeed the 68-kDa protein brought down by GST-14-3-3γ from mitotic extract ( Fig. 2b ). GFP-14-3-3γ and Myc–Plk1 were also coimmunoprecipitated from cells transfected with these proteins ( Supplementary Fig. S2a ). At endogenous levels, the two proteins were coimmunoprecipitated from mitotic but not interphase cell extracts ( Fig. 2c ). Among seven 14-3-3 members analysed, Plk1 had the highest affinity for the γ-subtype ( Fig. 2d ), indicating that Plk1 was likely to be a genuine binding partner of 14-3-3γ during mitosis. 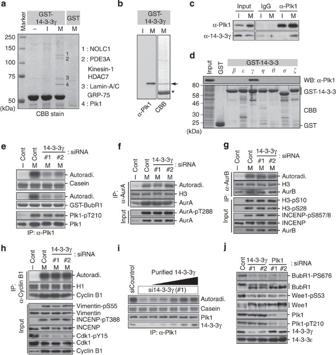Figure 2: 14-3-3γ binds to Plk1 and stimulates its catalytic activity. (a,b) Identification of proteins bound to GST-14-3-3γ specifically in mitotic extract. Mitosis- and 14-3-3γ-specific binding proteins (bands 1-4) are shown to the right (a). The presence of Plk1 was also checked by immunoblotting with anti-Plk1 (b). An asterisk or arrow indicates the position of GST-14-3-3γ or Plk1, respectively (b). (c) IP with anti-Plk1 from interphase (I) or mitotic (M) HeLa cell extract. The same amount of mouse IgG was used as a negative control. (d) GST pull-down assays using each subtype of GST-14-3-3 proteins form mitotic cell extract. (e–i) The effect of 14-3-3γ silencing on catalytic activities of mitotic kinases. Anti-Plk1 (e,i), anti-AurA (f), anti-AurB (g) or anti-Cyclin B1 immunoprecipitates (h) were subjected to IP kinase assays. Each immunoprecipitates and cell lysates (input) were also subjected to immunoblotting. Inf, 8–128 ng μl−1of purified 14-3-3γ was added in mitotic extract before IP. (j) The effects of 14-3-3γ or Plk1 depletion on intracellular phosphorylations. Figure 2: 14-3-3γ binds to Plk1 and stimulates its catalytic activity. ( a , b ) Identification of proteins bound to GST-14-3-3γ specifically in mitotic extract. Mitosis- and 14-3-3γ-specific binding proteins (bands 1-4) are shown to the right ( a ). The presence of Plk1 was also checked by immunoblotting with anti-Plk1 ( b ). An asterisk or arrow indicates the position of GST-14-3-3γ or Plk1, respectively ( b ). ( c ) IP with anti-Plk1 from interphase (I) or mitotic (M) HeLa cell extract. The same amount of mouse IgG was used as a negative control. ( d ) GST pull-down assays using each subtype of GST-14-3-3 proteins form mitotic cell extract. ( e – i ) The effect of 14-3-3γ silencing on catalytic activities of mitotic kinases. Anti-Plk1 ( e , i ), anti-AurA ( f ), anti-AurB ( g ) or anti-Cyclin B1 immunoprecipitates ( h ) were subjected to IP kinase assays. Each immunoprecipitates and cell lysates (input) were also subjected to immunoblotting. In f , 8–128 ng μl −1 of purified 14-3-3γ was added in mitotic extract before IP. ( j ) The effects of 14-3-3γ or Plk1 depletion on intracellular phosphorylations. Full size image After treatment with 14-3-3γ-specific siRNA, we then evaluated the catalytic activities of mitotic kinases in immunoprecipitates. Depletion of 14-3-3γ attenuated mitotic Plk1 activity towards casein or a GST-BubR1 fragment ( Fig. 2e ), whereas we observed only marginal changes in the activities of AurA ( Fig. 2f ), AurB ( Fig. 2g ), or Cdk1 ( Fig. 2h ). The reduction of Plk1 activity was reverted by the addition of purified 14-3-3γ to the immunoprecipitation (IP) lysate ( Fig. 2i ), suggesting that Plk1 binding to 14-3-3γ stimulated its catalytic activity. Remarkably, however, the silencing of 14-3-3γ had little impact on the phosphorylation status of Plk1–Thr210 in this assay ( Fig. 2e ). Next, we analysed the effect of 14-3-3γ-depletion in mitotic cells. Like Plk1 depletion, 14-3-3γ depletion reduced Plk1-induced phosphorylation of BubR1-Ser676 (ref. 24 ) and Wee1-Ser53 (ref. 25 ) ( Fig. 2j ). However, we observed no significant change in Plk1–Thr210 phosphorylation between control cells and 14-3-3γ-depleted cells. Collectively, these data suggested that 14-3-3γ specifically enhances Plk1 activity through a mechanism distinct from Plk1–Thr210 phosphorylation. Plk1–14-3-3γ interaction requires Plk1–Ser99 phosphorylation To examine the binding mode of the two proteins, we purified GST–Plk1 from insect cells and 14-3-3γ from Escherichia coli : GST–Plk1 was already phosphorylated at several sites including Thr210 in insect cells ( Supplementary Fig. S2b ). GST pull-down assays revealed a direct interaction between the two purified proteins, Plk1 and 14-3-3γ ( Supplementary Fig. S2b ). Remarkably, treatment of GST–Plk1 with λ protein phosphatase (λPPase) completely abolished the binding between the two proteins ( Supplementary Fig. S2b ). Thus, we mutated reported Plk1 phosphorylation sites, Ser137, Thr210 (ref. 26 ) and/or Ser326 (ref. 27 ) to Ala and then transfected cells with these Plk1 mutants. However, even mutation of all three sites (3A) did not inhibit the binding to GST-14-3-3γ ( Supplementary Fig. S2c ). As the N-terminal portion (residues 1–201) of Plk1 was sufficient for the binding to 14-3-3γ ( Fig. 3a ), we constructed a series of Plk1 fragments (1–371) mutated at Ser or Thr residues within 1–201. As shown in Fig. 3b , Ala mutation at Ser99 specifically abolished the binding to GST-14-3-3γ, suggesting that Ser99 was the most likely candidate phosphorylation site required for 14-3-3γ binding. 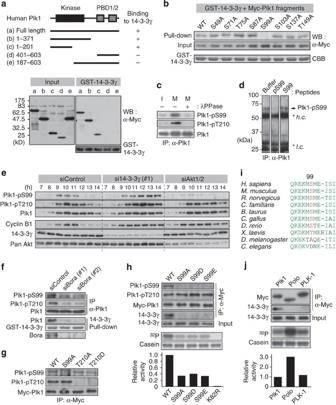Figure 3: Ser99 is a novel phosphorylation site required for Plk1 binding to 14-3-3γ. (a,b) The indicated Myc–Plk1 fragments were transiently expressed in HeLa cells. Inb, Myc–Plk1 fragments (residues 1–371) were mutated at the indicated Ser/Thr to Ala. Each mitotic extract was subjected to GST pull-down assays using GST-14-3-3γ (c) Endogenous Plk1 was immunoprecipitated from interphase (I) or mitotic (M) extract. Before the immunoblotting, the immunoprecipitates were treated with or without λPPase. (d) Specificity of anti-Plk1-pS99 was analysed by the peptide competition assays. The position of heavy (h.c.) or light (l.c.) chain of anti-Plk1 is also indicated. (e) The effect of 14-3-3γ or Akt1/2 silencing on cell-cycle progression after DTB synchronization. (f) The effect of Bora silencing on Plk1 phosphorylation. (g–j) Myc–Plk1 WT or its variant was induced by the addition of doxycycline (Dox) in Tet-On HeLa cells (g,h). Inj, Myc-tagged human Plk1 (WT), fly Polo or nematode PLK1 was transiently introduced in HeLa cells. Each anti-Myc immunoprecipitate from mitotic cells was subjected to immunoblotting or IP kinase assays. Fold activation relative to Plk1 WT is shown in the graph. The alignment of Plk1 protein sequences around Ser99 is shown ini. Figure 3: Ser99 is a novel phosphorylation site required for Plk1 binding to 14-3-3γ. ( a , b ) The indicated Myc–Plk1 fragments were transiently expressed in HeLa cells. In b , Myc–Plk1 fragments (residues 1–371) were mutated at the indicated Ser/Thr to Ala. Each mitotic extract was subjected to GST pull-down assays using GST-14-3-3γ ( c ) Endogenous Plk1 was immunoprecipitated from interphase (I) or mitotic (M) extract. Before the immunoblotting, the immunoprecipitates were treated with or without λPPase. ( d ) Specificity of anti-Plk1-pS99 was analysed by the peptide competition assays. The position of heavy (h.c.) or light (l.c.) chain of anti-Plk1 is also indicated. ( e ) The effect of 14-3-3γ or Akt1/2 silencing on cell-cycle progression after DTB synchronization. ( f ) The effect of Bora silencing on Plk1 phosphorylation. ( g – j ) Myc–Plk1 WT or its variant was induced by the addition of doxycycline (Dox) in Tet-On HeLa cells ( g , h ). In j , Myc-tagged human Plk1 (WT), fly Polo or nematode PLK1 was transiently introduced in HeLa cells. Each anti-Myc immunoprecipitate from mitotic cells was subjected to immunoblotting or IP kinase assays. Fold activation relative to Plk1 WT is shown in the graph. The alignment of Plk1 protein sequences around Ser99 is shown in i . Full size image In order to examine Plk1–Ser99 phosphorylation in vivo , we produced a phosphoepitope-specific antibody by immunizing guinea pigs with a phosphopeptide comprising phosphorylated Ser99 and its surrounding sequence [28] , [29] . This antibody reacted with a band of about 68 kDa, corresponding to endogenous Plk1 immunoprecipitated from mitotic cells but not from interphase cells ( Fig. 3c ). This immunoreactivity was abolished by pretreatment of the anti-Plk1 immunoprecipitate with λPPase ( Fig. 3c ) or preincubation of the phosphoepitope-specific antibody with the phosphorylated version of the S99 peptide ( Fig 3d ), confirming the specificity of the anti-Plk1-pS99 antibody. As this antibody could not be used for immunocytochemistry, we analysed the in vivo phosphorylation of Plk1 by western blotting experiments after anti-Plk1 IP. As shown in Fig. 3e , Plk1–Ser99 phosphorylation was detected mainly from 9 h to 11 h after the release from a second thymidine block. This pattern was similar to the changes in Cyclin B1 levels ( Fig. 3e ), suggesting that Plk1–Ser99 phosphorylation occurs especially during early mitosis. In 14-3-3γ-depleted cells, Plk1 phosphorylation on Ser99 and Thr210 were prolonged after the release from the second thymidine block ( Fig. 3e ). As the destruction of Cyclin B1 was also impaired in these cells ( Fig. 3e ), the prolongation was likely due to a prometaphase/metaphase-like arrest ( Fig. 1 ). The level of Plk1–Ser99 phosphorylation was elevated at about the same time as Plk1–Thr210 phosphorylation ( Fig. 3e ). As initial Plk1–Thr210 phosphorylation largely depends on the protein level of Bora [10] , [11] , which peaks at the G2/M transition [30] , [31] , we examined whether Bora also regulates Plk1–Ser99 phosphorylation. As shown in Fig. 3f , silencing of Bora indeed reduced the level of Plk1 phosphorylation not only at Thr210, but also at Ser99. Here the figure also shows that Bora depletion reduces the interaction between Plk1 and 14-3-3γ. This is in good agreement with the earlier data showing Ser99 phosphorylation mediates interaction with 14-3-3γ ( Fig. 3b ). To evaluate the relationship between phosphorylations at these two sites, we generated Tet-ON HeLa cell lines expressing Myc–Plk1 WT or corresponding mutants carrying Ala (A), Asp (D) or Glu (E) at Ser99 or Thr210. As shown in Fig. 3g , Thr210 mutation had only marginal effects on Ser99 phosphorylation status and vice versa. Thus, these results suggested that Plk1–Ser99 phosphorylation occurs independently of Plk1–Thr210 phosphorylation but that Bora controls both phosphorylation processes. 14-3-3γ interaction stimulates Plk1 activity Using the above Tet-On HeLa cell lines, we directly evaluated the function of mitotic Plk1–Ser99 phosphorylation. IP with anti-Myc revealed that mutations of Ser99 reduced both 14-3-3γ binding and catalytic activity without affecting the phosphorylation status of Plk1–Thr210; S99D or S99E behaved like S99A ( Fig. 3h ). Unlike the situation with WT protein, the residual activity of S99A could not be stimulated by addition of 14-3-3γ to the IP extract ( Supplementary Fig. S3a ). Interestingly, Ser99 is conserved among vertebrates but not in fly or nematode Plk1 ( Fig. 3i ), suggesting that Plk1 regulation by 14-3-3γ was acquired during vertebrate evolution. Indeed, D. melanogaster (Polo) or Caenorhabditis elegans (PLK1) orthologues, both of which lack Ser99, do not bind to 14-3-3γ, but are nevertheless catalytically active when expressed in mitotic HeLa cells ( Fig. 3j ). Also, these results support the conclusion that human Plk1–Ser99 is the target (phosphorylation) site required for 14-3-3γ binding. To assess the role of Ser99 phosphorylation on endogenous Plk1 substrates, we replaced endogenous Plk1 with siRNA-resistant Myc–Plk1 WT or mutant proteins by transfection of Tet-ON cells with Plk1-specific siRNA (siPlk1). As Ser99 mutation ( Fig. 4a and Supplementary Fig. S3b ) or 14-3-3γ depletion ( Fig. 4b ) had little impact on Plk1 localization in mitosis, Plk1 phosphorylation at Ser99 and binding to 14-3-3γ are dispensable at least for Plk1 recruitment to centrosomes and KTs. On the other hand, the replacement of WT Plk1 by the S99A mutant reduced Plk1-induced phosphorylation of BubR1-Ser676 and Wee1-Ser53 in mitotic cells ( Fig. 4c ). Together with the data obtained by IP kinase assays ( Fig. 3h ), these results suggested that Plk1 phosphorylation at Ser99 stimulates the catalytic activity of Plk1. 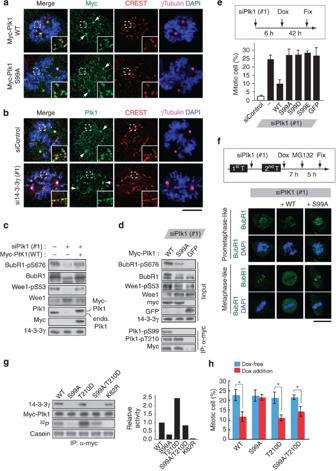Figure 4: Plk1–Ser99 phosphorylation is indispensable for Plk1 activation pathway via 14-3-3γ. (a) Myc–Plk1 WT and S99A were introduced in Tet-On HeLa cells and then stained with anti-Myc (green), anti-γ-tubulin (magenta) and CREST (red). (b) The effect of 14-3-3γ silencing on subcellular localization of endogenous Plk1. Arrows indicate the position of centrosomes. (c,d) The evaluation of mitotic protein phosphorylation after the replacement of endogenous Plk1 with exogenous Myc–Plk1, using the indicated Tet-On HeLa cell line. Owing to silent mutation on the gene coding each Myc–Plk1, the induced messenger RNA is resistant to Plk1 siRNA target sequence #1 (siPlk1, #1). Tet-On HeLa cells expressing GFP were used as a negative control (d). (e,h) The evaluation of mitotic index after the replacement. Inh, Tet-On cells incubated without doxycycline after the treatment with siPlk1 (#1) are used as negative controls. (f) The effects of the replacement on KT-associated BubR1. Scale bars, 10 μm. (g) Each Myc–Plk1 construct was immunoprecipitated from mitotic Tet-On cells and then subjected to immunoblotting or IP kinase assays. Figure 4: Plk1–Ser99 phosphorylation is indispensable for Plk1 activation pathway via 14-3-3γ. ( a ) Myc–Plk1 WT and S99A were introduced in Tet-On HeLa cells and then stained with anti-Myc (green), anti-γ-tubulin (magenta) and CREST (red). ( b ) The effect of 14-3-3γ silencing on subcellular localization of endogenous Plk1. Arrows indicate the position of centrosomes. ( c , d ) The evaluation of mitotic protein phosphorylation after the replacement of endogenous Plk1 with exogenous Myc–Plk1, using the indicated Tet-On HeLa cell line. Owing to silent mutation on the gene coding each Myc–Plk1, the induced messenger RNA is resistant to Plk1 siRNA target sequence #1 (siPlk1, #1). Tet-On HeLa cells expressing GFP were used as a negative control ( d ). ( e , h ) The evaluation of mitotic index after the replacement. In h , Tet-On cells incubated without doxycycline after the treatment with siPlk1 (#1) are used as negative controls. ( f ) The effects of the replacement on KT-associated BubR1. Scale bars, 10 μm. ( g ) Each Myc–Plk1 construct was immunoprecipitated from mitotic Tet-On cells and then subjected to immunoblotting or IP kinase assays. Full size image Plk1–Ser99 phosphorylation is required for mitotic progression The mitotic arrest caused by Plk1 silencing was largely overcome by the expression of Plk1 WT, but not Plk1 mutated at Ser99 ( Fig. 4e ). In all experiments, mutations of Ser99 to Ala or Asp/Glu produced similar results ( Figs 3h , 4e ; also see Fig. 4a and Supplementary Fig. S3b ), suggesting that S99D or S99E did not mimic Plk1–Ser99 phosphorylation. As judged by BubR1 signals on KTs in metaphase-like cells, SAC activation was also reverted by the induction of Plk1 WT but not S99A ( Fig. 4f ). Thus, Plk1 phosphorylation at Ser99 is required for proper mitotic progression from metaphase to anaphase. In order to examine more precisely how 14-3-3γ modulates mitotic Plk1 function, we searched for a Plk1 mutant that would display near-WT activity but lack 14-3-3γ binding. As mutation of Thr210 to Asp (T210D) strongly elevates the catalytic activity of Plk1 in mitotic cells (WT versus T210D in Fig. 4g ), we combined this mutation with Ala mutation at Ser99. As shown in Fig. 4g , the S99A/T210D double mutant had lost 14-3-3γ binding but showed activity almost equivalent to WT protein in mitotic cells, indicating that the Ser99 mutation diminished the catalytic activity not only of WT Plk1, but also of the T210D mutant (see WT versus S99A and T210D versus S99A/T210D in Fig. 4g ). Unlike induction of S99A, induction of S99A/T210D was able to overcome the mitotic arrest induced by Plk1 silencing ( Fig. 4h ), suggesting that 14-3-3γ regulates mitotic Plk1 function primarily through the stimulation of Plk1 activity. As Plk1 was also reported to have important roles in entry into mitosis after checkpoint recovery [10] , [11] , we analysed the mitotic index after release from DTB-induced arrest. Strong silencing of Plk1 expression (siPlk1, 3′-untranslated region) induced a delay in mitotic entry, whereas weaker Plk1 depletion (siPlk1, #1) had only a marginal effect ( Fig. 5a ). This delay in mitotic entry was reverted by the expression of S99A, as well as WT Plk1 but not a Thr210-phospho-blocking mutant (T210A) or an ATP-binding-site mutant (K82R; Fig. 5c ). Importantly, these latter mutants almost completely lacked catalytic activity, whereas Plk1–S99A activity was weak but detectable ( Supplementary Fig. S3c ; also see Fig. 3h ). Similar effects on the kinetics of mitotic entry were observed when using nocodazole to arrest cells through SAC activation ( Supplementary Fig. S3d ). Next, we examined the functionality of Plk1 mutants during centrosome separation. Monopolar spindle formation was increased by strong Plk1 depletion (3′-untranslated region) but only marginally by partial depletion (#1; Fig. 5a ). This monopolar spindle formation was reverted by the induction of S99A, as well as WT but not T210A or K82R versions of Plk1 ( Fig. 5e ). Consistent with these results, 14-3-3γ depletion had only marginal effects on the kinetics of mitotic entry after DTB-induced arrest ( Fig. 1b ) or the extent of bipolar spindle formation ( Fig. 5f ). These results suggested that Plk1 binding to 14-3-3γ through Plk1–Ser99 phosphorylation is dispensable for mitotic entry after checkpoint recovery, as well as for centrosome separation. They support and extend a previous study demonstrating that different mitotic functions of Plk1 show differential sensitivity to Plk1 regulatory mechanisms [32] . 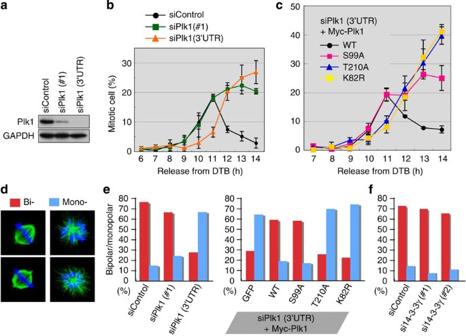Figure 5: Plk1–Ser99 phosphorylation is dispensable for mitotic entry after release from a second block. (a) The evaluation of Plk1 silencing using each target sequence of Plk1 (#1 or 3′-untranslated region (UTR)). (b) The effect of Plk1 silencing on mitotic entry after DTB synchronization. (c) The evaluation of mitotic index after the replacement. (d) The effect of Plk1 silencing on spindle bipolarity. Examples of monopolar or bipolar spindle formation are shown in the left. (e,f) The effect of the replacement with the indicated Plk1 (e) or 14-3-3γ silencing (f) on bipolar spindle formation. Data were obtained from two independent experiments (n>100;d–f). GAPDH, glyceraldehyde 3-phosphate dehydrogenase. Figure 5: Plk1–Ser99 phosphorylation is dispensable for mitotic entry after release from a second block. ( a ) The evaluation of Plk1 silencing using each target sequence of Plk1 (#1 or 3′-untranslated region (UTR)). ( b ) The effect of Plk1 silencing on mitotic entry after DTB synchronization. ( c ) The evaluation of mitotic index after the replacement. ( d ) The effect of Plk1 silencing on spindle bipolarity. Examples of monopolar or bipolar spindle formation are shown in the left. ( e , f ) The effect of the replacement with the indicated Plk1 ( e ) or 14-3-3γ silencing ( f ) on bipolar spindle formation. Data were obtained from two independent experiments ( n >100; d–f ). GAPDH, glyceraldehyde 3-phosphate dehydrogenase. Full size image PI3K pathway inhibition impairs Plk1–Ser99 phosphorylation As Akt was reported to participate in mitotic control [33] , [34] , we examined the participation of the PI3K–Akt pathway in this Plk1 novel activation pathway. As shown in Figs 6a and 3e , the treatment with Akt1- and Akt2-specific siRNAs (siAkt1/2) decreased the level of Plk1 phosphorylation at Ser99, but not at Thr210. Double knockdown also reduced the interaction between Plk1 and 14-3-3γ ( Fig. 6a ). We observed only marginal effects in the case of silencing of single Akt isoforms ( Fig. 6a ), suggesting that Akt1 or Akt2 can compensate for each other at least in these assays. Consistent with the data obtained by double knockdown of Akt1/2, the treatment of cells with MK-2206 (refs 35 , 36 ), API-2 (ref. 37 ) (Akt inhibitors that suppress Akt activation processes including Akt–Ser473 phosphorylation), wortmannin or LY294002 (the inhibitors of PI3K upstream of Akt) reduced both Plk1–Ser99 phosphorylation and the interaction between Plk1 and 14-3-3γ ( Supplementary Fig. S4a ). IP kinase assays also revealed that treatment with siAkt1/2-reduced Plk1 activity ( Fig. 6b ). 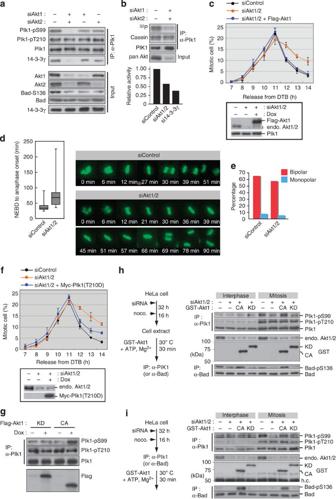Figure 6: Akt participates in Plk1 activation process via 14-3-3γ by regulating Plk1–Ser99 phosphorylation. (a,b) The effect of Akt silencing on Plk1 phosphorylation, Plk1 interaction with 14-3-3γ (a) and Plk1 catalytic activity (b). (c, f) Using Tet-On HeLa cells expressing Flag-Akt1 WT (c) or Myc–Plk1 T210D (f), we performed the combination of DTB synchronization and the treatment with Akt1- and Akt2-specific siRNAs (siAkt1/2) as described in Hirotaet al.16Just after release from second thymidine block, the cells were cultured with (+) or without (−) doxycycline in the medium. Each protein level was checked by the immunoblotting with anti-Akt and anti-Plk1 (c) or anti-Myc (f). (d) Live-cell imaging analyses using H2B-GFP-expressing HeLa cells (n≥130 from two independent experiments). (e) The effect of Akt silencing on bipolar spindle formation. (g) KD or CA Flag-Akt1 was introduced in Tet-ON HeLa cells, and then mitotic phosphorylation of Plk1 was evaluated. (h,i)In vitroAkt kinase assays using depleted/reconstituted HeLa cell extracts (h) or anti-Plk1 immunoprecipitates (i) were performed as described in ‘Methods’. These results indicate that the effects of PI3K–Akt pathway inhibition on Plk1 function ( Fig 6a ) closely resemble those of 14-3-3γ depletion ( Fig. 2e ) or Plk1–Ser99 mutation ( Fig. 3h ). Figure 6: Akt participates in Plk1 activation process via 14-3-3γ by regulating Plk1–Ser99 phosphorylation. ( a , b ) The effect of Akt silencing on Plk1 phosphorylation, Plk1 interaction with 14-3-3γ ( a ) and Plk1 catalytic activity ( b ). ( c, f ) Using Tet-On HeLa cells expressing Flag-Akt1 WT ( c ) or Myc–Plk1 T210D ( f ), we performed the combination of DTB synchronization and the treatment with Akt1- and Akt2-specific siRNAs (siAkt1/2) as described in Hirota et al. [16] Just after release from second thymidine block, the cells were cultured with (+) or without (−) doxycycline in the medium. Each protein level was checked by the immunoblotting with anti-Akt and anti-Plk1 ( c ) or anti-Myc ( f ). ( d ) Live-cell imaging analyses using H2B-GFP-expressing HeLa cells ( n ≥130 from two independent experiments). ( e ) The effect of Akt silencing on bipolar spindle formation. ( g ) KD or CA Flag-Akt1 was introduced in Tet-ON HeLa cells, and then mitotic phosphorylation of Plk1 was evaluated. ( h , i ) In vitro Akt kinase assays using depleted/reconstituted HeLa cell extracts ( h ) or anti-Plk1 immunoprecipitates ( i ) were performed as described in ‘Methods’. Full size image PI3K pathway inhibition impairs mitotic progression As described above [16] , we again combined siRNA transfection with DTB synchronization; here to study cell-cycle progression in the absence of Akt1/2. In comparison with cells treated with siControl, siAkt1/2 produced only marginal changes in the timing of mitotic entry and the height of the mitotic index peak, but the decline in mitotic index after release from a second thymidine block was clearly less efficient ( Fig. 6c ). This phenotype could be reversed by the induction of Flag-Akt1 WT expression ( Fig. 6c ), indicating that it was specific to Akt1/2 depletion rather than an off-target effect. Consistent with the above observations, the treatment of cells with a PI3K or Akt inhibitor showed similar phenotypes ( Supplementary Fig. S4b ). Moreover, as shown in Fig. 6d (see also Supplementary Movies 3 and 4 ), the duration from nuclear envelope breakdown to anaphase onset was much longer in cells treated with siAkt1/2 (mean of 92 min) than in siControl (mean of 40 min). Like 14-3-3γ silencing ( Fig. 5f ) or the replacement of WT Plk1 by the S99A mutant ( Fig. 5e ), Akt1/2 depletion resulted in marginal effects on the extent of bipolar spindle formation ( Fig. 6e ). Importantly, expression of a hyperactive Plk1 mutant (T210D) could compensate for knockdown of Akt1/2 ( Fig. 6f ) and, conversely, the induction of a constitutively active (CA) Akt mutant enhanced the mitotic phosphorylation of Plk1–Ser99 ( Fig. 6g ). These results suggest that the PI3K–Akt pathway participates in a Plk1 activation process by controlling Plk1–Ser99 phosphorylation, a regulatory step necessary for the interaction between Plk1 and 14-3-3γ. We then performed in vitro kinase assays, using a Plk1 kinase-dead (KD) mutant purified from bacteria as a substrate. As reported previously [10] , [11] , AurA phosphorylates Plk1 in a Bora-dependent manner ( Supplementary Fig. S5a ). On the other hand, Plk1 purified from bacteria did not appear to be a good in vitro substrate for Akt, regardless of Bora ( Supplementary Fig. S5b ). However, the regulation of mitotic Plk1 phosphorylation in vivo is known to be complex in that Bora or INCENP are required for Plk1–Thr210 phosphorylation by AurA [10] , [11] or AurB [12] , respectively. These findings led us to postulate that additional factor(s) might be required for Plk1–Ser99 phosphorylation. To examine this possibility, two types of experiments were performed. First, we examined phosphorylation of Plk1 in HeLa extracts that had been depleted of endogenous Akt1/2 and reconstituted by recombinant Akt. Upon back-addition of a CA form of GST–Akt1, the phosphorylation of endogenous Plk1 at Ser99 was elevated in the mitotic extract but not in the interphase extract, whereas phosphorylation of endogenous Bad at Ser136 [38] , [39] (a control Akt substrate) was observed in both interphase and mitotic extracts ( Fig. 6h ). In a second type of experiment, we used immunoprecipitated Plk1 rather than recombinant Plk1 as an in vitro substrate for Akt. Using anti-Plk1 immunoprecipitates from mitotic cells, we also observed that Plk1–Ser99 phosphorylation was induced by GST–Akt1 CA, but not KD ( Fig. 6i ). In contrast, no such phosphorylation was detected when using anti-Plk1 immunoprecipitates from interphase cells ( Fig. 6i ). Similar results were obtained when analysing exogenous Myc–Plk1 immunoprecipitated from mitotic cells ( Supplementary Fig. S5c ). Collectively, these in vitro kinase assays strongly suggest that Plk1–Ser99 phosphorylation requires not only Akt activity but also a factor(s) that associate with Plk1 in a mitosis-specific fashion. In this study, we characterize a novel Plk1 activation pathway distinct from Plk1–Thr210 phosphorylation. Our model is summarized in Fig. 7 . Bora binding to Plk1 is thought to induce a conformational change in Plk1 [10] , which in turn favours Plk1 phosphorylation not only at Thr210 but also at Ser99. Plk1–Ser99 phosphorylation occurs independently of Plk1–Thr210 phosphorylation, but largely depends on the catalytic activity of Akt downstream of PI3K. Ser99 phosphorylation induces the recruitment of 14-3-3γ to Plk1, which, together with Thr210 phosphorylation, elevates the catalytic activity of Plk1. 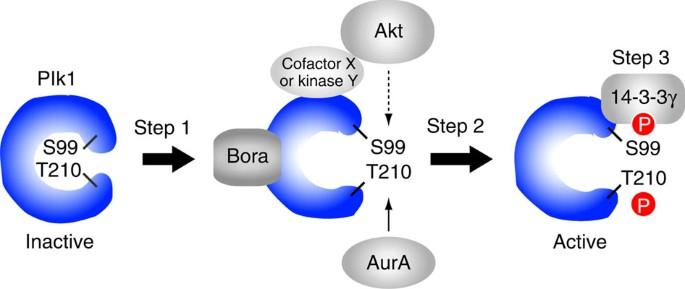Figure 7: A proposed model of Plk1 activation.  Figure 7: A proposed model of Plk1 activation. Full size image AurA was reported to directly phosphorylate Thr210 on Plk1 in a Bora-dependent manner [10] , [11] , and our in vitro results support this conclusion ( Supplementary Fig. S5a ). The regulation of Plk1–Ser99 phosphorylation may follow a similar pattern or be more complex. Neither Plk1 purified from bacteria ( Supplementary Fig. S5b ) nor Plk1 immunoprecipitated from interphase cells ( Fig. 6h ) was a good substrate for Akt, whereas Plk1 precipitated from mitotic cells could be phosphorylated at Ser99 in vitro in a manner that required the catalytic activity of Akt ( Fig. 6h and Supplementary Fig. S5c ). Thus, much like Plk1–Thr210 phosphorylation by AurA [10] , [11] or AurB [12] , Plk1–Ser99 phosphorylation by Akt is likely to require additional, as yet unidentified protein(s) that associate with Plk1 in a mitosis-specific manner. One possibility is that a mitotic cofactor turns Plk1 into a direct Akt substrate. Alternatively, Akt may phosphorylate and activate a Ser99-specific kinase that specifically associates with Plk1 during mitosis or Akt may regulate cofactor that exposes Ser99 on Plk1 for phosphorylation by another kinase. Thus, the detailed mechanism underlying the Akt-dependent regulation of Plk1–Ser99 phosphorylation remains to be unravelled. In addition, we note that the PI3K–Akt pathway may not be the sole route to control Plk1 phosphorylation at Ser99; in fact, the phenotypes observed after interference with the PI3K–Akt pathway ( Fig. 6c and Supplementary Fig. S4b ) are slightly milder than those seen after 14-3-3γ depletion ( Fig. 1b ) or the replacement of endogenous Plk1 by the S99A mutant ( Fig. 5c ). Thus, we conclude that Plk1–Ser99 phosphorylation is largely under the control of the PI3K–Akt pathway but likely to require additional regulators. Why is Plk1 activation pathway via 14-3-3γ only required for some but not all Plk1 functions? One possible explanation is that different functions require different thresholds of Plk1 activity. Consistent with this idea, the phenotypes of Plk1 silencing were found to depend on residual Plk1 protein and/or activity. Strong depletion of Plk1 led cells to arrest with monopolar spindles likely due to inhibition of centrosome maturation/separation ( Fig. 5a ), and it also impaired entry into mitosis after release from a DTB ( Fig. 5a ). However, moderate depletion did not impair these early mitotic functions ( Fig. 5a ). Instead, moderate depletion induced a SAC-dependent, prometaphase/metaphase-like arrest likely due to impaired KT–MT attachments ( Fig. 5a ). Similarly, an earlier study found that polo-box-domain mediated targeting of Plk1 was indispensable for chromosome congression but not strictly required for centrosome maturation and bipolar spindle formation [32] . In the present study, we found that Plk1 catalytic activity was reduced by the inhibition of Plk1 activation thorough Ser99 phosphorylation and 14-3-3γ binding ( Figs 2e , 3f , and 6b ), while interference with Plk1–Thr210 phosphorylation completely abolished all activity ( Supplementary Fig. S4c ). Thus, we propose that maximal Plk1 activation through both Ser99 phosphorylation/14-3-3γ binding and Plk1–Thr210 phosphorylation is required for proper and complete KT–MT attachments and the transition from metaphase to anaphase. In addition, it is possible that Plk1–Ser99 phosphorylation is particularly critical for Plk1 functionality at KTs. In support of this possibility, we note that the phenotype of perturbation of the Plk1 activation pathway via 14-3-3γ resembles that of repression of Plk1 function at KTs [32] , [40] . In conclusion, the present study documents the functional importance of Plk1–Ser99 phosphorylation and 14-3-3γ in proper progression from metaphase to anaphase and paves the way for future studies evaluating the relationship between Plk1 activity and chromosomal stability. The mechanism by which the PI3K–Akt pathway controls Plk1–Ser99 phosphorylation will be addressed in the future. Antibodies Guinea Pig polyclonal anti-Plk1-pS99 antibody was produced with a phosphopeptide pS99 (CQKEKM-S[PO3H2]-MEISI; Peptide Institute Inc., Osaka, Japan), as previously described [28] , [29] . In the competition assay ( Fig. 3d ), anti-Plk1-pS99 was preincubated with 50 ng ml −1 of the phosphopeptide pS99 or the corresponding non-phosphorylated peptide S99 at 4 °C for 1 h. Rat monoclonal anti-Histone H3 pSer28 (ref. 15 ), anti-INCENP pThr388 (ref. 40 ), mouse mononclonal anti-Vimentin pSer55 (ref. 41 ), rabbit polyclonal anti-Wee1 pSer53 (ref. 25 ), anti-INCENP pSer857/pSer858 (ref. 40 ), anti-Bora [30] and anti-BubR1 pSer676 (ref. 24 ) were described. Antibodies from commercial sources were as follows: mouse anti-Plk1 (F-8), anti-α-tubulin (DM1A), anti-Bad (C-7) and rabbit anti-14-3-3γ (C-16) from Santa Cruz Biotechnology (Santa Cruz, CA); rabbit anti-Cdk1 pY15 (10A11), anti-pan Akt (40D4), anti-Akt1 (C73H10), anti-Akt2 (D6G4), anti-Bad (D24A9), anti-Bad pSer136 (D25H8), anti-Wee1 and HRP-conjugated anti-GAPDH from Cell Signaling Technology (Beverly, MA); mouse anti-Plk1 pThr210 (2A3) from Abcam (Cambridge, UK); mouse anti-14-3-3γ (CG31-2B6) and anti-Myc (4A6) from Millipore (Bedford, MA); mouse anti-γ-tubulin (GTU-88), anti-Vimentin (V9), anti-Flag (M2) and rabbit anti-INCENP from Sigma (St Louis, MO); mouse anti-Cdk1, anti-Aurora A and anti-Aurora B from BD Transduction Laboratories (San Diego, CA); rabbit anti-Mad2 from Covance (NJ, USA); mouse anti-BubR1 (8G1) and rabbit anti-histone H3 pSer10 from Medical & Biological Laboratories Co., Ltd. (Nagoya, Japan); and CREST antiserum from Fitzgerald Industries International (North Acton, MA). Cell culture and synchronization We established Tet-On HeLa cells expressing Myc-tagged Plk1 or 3xFlag-tagged Akt1 as described previously [42] . Plk1 complementary DNA (cDNA) was mutated at four (silent) bases to make the transcript resistant to Plk1 siRNA-#1. Construction of KD [43] or constitutive-active (CA; residues 118-end containing Ser473 mutation to Asp) Akt1 was performed with KOD-Plus-Mutagenesis Kit (TOYOBO Co. Ltd., Osaka, Japan). For expression of Plk1 or Akt1, Tet-ON HeLa cells were incubated with 300 ng ml −1 of doxycycline (Sigma, St Louis, MO). Cells were cultured in a 5% CO 2 atmosphere in DME (Invitrogen) supplemented with 10% FBS. Thymidine (2 mM) was obtained from Wako (Osaka, Japan). MG132 (10 μM) and nocodazole (100 ng ml −1 ) were obtained from Merck (Darmstadt, Germany). After the treatment with nocodazole, interphase or mitotic HeLa cells were prepared as described [44] . For combination of DTB synchronization and siRNA-mediated knockdown, siRNA was transfected immediately after release of first thymidine block [16] . Mitotic index was evaluated as described [13] , [42] . Immunofluorescence and immunoprecipitation Cells were fixed with 3% formaldehyde in PHEM buffer (60 mM Pipes, 25 mM Hepes, 10 mM EGTA and 2 mM MgSO 4 , pH 7.0) at room temperature for 20 min, and permeabilized with 0.05% Triton X-100 in PBS. Then, Cells were stained with the indicated antibodies and 4',6-diamidino-2-phenylindole as described [42] . Immunoblotting and immunoprecipitation were performed as described elsewhere [13] , [42] . Live-cell imaging Histone H2B-GFP-expressing HeLa cell was kindly provided by Hirota et al. [16] Cells were treated with a combination of DTB synchronization and siRNA transfection [16] . From 6 to 15 h after the release from second thymidine block, images were acquired every 3 min on an Olympus IX71 microscope (Tokyo, Japan). GFP signal was acquired at each time point with a 3-ms exposure time. Experiments were performed in a temperature-controlled chamber, which was maintained at 37 °C with a humidified atmosphere of 5% CO 2 in air. Metamorph software (Molecular Devices, Downingtown, PA) was used for acquisition and analysis. The results are displayed as box-and-whisker plots; boxes represent 25–75% of the cell, the line with the box indicates the median and whiskers represent the 5th and 95th percentiles, respectively. Transfection The cDNAs for D. melanogaster Polo and C. elegan s PLK1 were obtained from DGRC (clone LD11851) and National Institute of Genetics (clone yk1383e06), respectively. Human Plk1 (including its mutants) and the above Plk1 orthologues were inserted into pCMV-Tag3B (Stratagene, La Jolla, CA). Plasmid transfection was performed with Lipofectamine LTX and PLUS Reagents according to the manufacturer’s protocol (Invitrogen, Carlsbad, CA). Protein purification We generated the recombinant baculovirus encoding the CA or KD [43] mutant of human Akt1 using a combination of the GATEWAY vector conversion system and the Bac-to-Bac baculovirus expression system (Invitrogen). GST-tagged human Plk1 and AurA were expressed in baculovirus-infected Sf9 cells [45] , [46] . GST-tagged Plk1 KD mutant (Asp194 mutation to Ala; D194A) and maltose binding protein (MBP)-tagged Bora were expressed in E. coli strain BL21 CodonPlus RP (Stratagene). GST-tagged 14-3-3 proteins [13] and BubR1 fragments (residues 641–720) were expressed in E. coli strain DH5α (Invitrogen). GST- or MBP-tagged proteins were purified through affinity chromatography with glutathione-sepharose 4B (GE Healthcare, Little Chalfont Buckinghamshire, UK) or amylose resin (New England Biolabs, Ipswich, MA), respectively. GST pull-down assays were performed as described [13] . In some experiments, GST was removed from GST-14-3-3γ by PreScission Protease (GE Healthcare). The dephosphorylation reaction was performed by the incubation with lambda protein phosphatase (λPPase) in the equipped buffer (New England Biolabs) for 60 min at 30 °C. Identification of proteins bound to GST-14-3-3γ Mitotic and interphase HeLa cells were treated with cell lysis buffer (20 mM Tris-Cl (pH 7.5), 150 mM NaCl, 2 mM β-glycerophosphate, 50 mM NaF, 1 mM Na 3 VO 4 , 2.5 mM sodium pyrophosphate, 2 mM EDTA, 1 mM EGTA and 1% Triton X-100) containing protease inhibitor cocktail (Nacalai, Kyoto, Japan) for 30 min at 4 °C. After centrifugation (17,000 g , 15 min), each cell extract (50 mg of total protein) was incubated with 100 μg of GST or GST-14-3-3γ for 2 h at 4 °C. After further centrifugation (17,000 g , 30 min), each mixture was rotated with 200 μl of glutathione-sepharose 4B beads (GE Healthcare) for 30 min at 4 °C. The beads were washed with 10 ml of ice-cold cell lysis buffer five times. GST-14-3-3γ was eluted in ice-cold buffer containing 20 mM reduced glutathione, 50 mM Tris-Cl (pH 8.8) and 150 mM NaCl. The eluted solution was concentrated with Amicon Ultra-10 K (Millipore) at 4 °C and then subjected to mass spectrometry analysis as follows: after SDS–polyacrylamide gel electrophoresis, bound proteins were processed using an in-gel trypsin digestion kit (Thermo Fisher Scientific, Waltham, MA), and the resulting peptides were analysed by 4800 Plus MALDI TOF/TOF Analyzer (AB Sciex, Foster City, CA). The mass spectrometric data were searched by the Mascot search engine (Matrix Science, Boston, MA) against SwissProt. IP kinase assays Each immunoprecipitate was incubated with 4 μg of casein (Roche Diagnostics, Mannheim, Germany), GST-BubR1 fragment (641–720 residues; for Plk1), histone H3 (Roche Diagnostics; for AurA and AurB) and histone H1 (Roche Diagnostics; for Cdk1) in 20 μl of reaction buffer (25 mM Tris-Cl (pH 7.5), 10 mM MgCl 2 , and 10 μM [γ- 32 P]ATP) at 30 °C for 10 (for Plk1 and Cdk1) or 30 (for AurA and AurB) min. In vitro kinase assay using purified proteins GST–Plk1 D194A (100 μg ml −1 ) was incubated with 20 μg ml −1 of GST–Akt1 CA or GST-AurA WT in the presence of MBP-Bora (25–400 μg ml −1 ) or MBP (400 μg ml −1 ) in 20 μl of reaction buffer (25 mM Tris-Cl (pH 7.5), 50 mM NaCl, 0.1 mM [γ- 32 P]ATP, 10 mM MgCl 2 , 0.5 mM EGTA, 0.5 mM DTT) at 30 °C for 10 min. In vitro kinase assays using HeLa cell extracts HeLa cells ( Fig. 6h ) or Tet-ON cells expressing Myc–Plk1 ( Supplementary Fig. S5c ) were transfected with control siRNA or siAkt1/2 as described above. Thirty two hours after the transfection with each set of siRNA, we added 100 nM nocodazole into the growth media. In the case of Tet-ON cell lines, we also added 300 ng ml −1 of doxycycline. Sixteen hours after the treatment with nocodazole, interphase or mitotic cells were collected as described [44] . Akt reconstitutions of cell extracts and kinase assays ( Fig. 6h ) were performed as follows. Interphase or mitotic HeLa cells (each ~2.5 × 10 6 cells) were incubated with 100 μl of cell lysis buffer on ice for 15 min. After centrifugation (17,000 g ) for 15 min at 4 °C, each supernatant (100 μl) was diluted with 400 μl of reaction buffer (25 mM Tris-Cl (pH 7.5), 75 mM NaCl, 10 mM MgCl 2 ). The above mixture was incubated with or without GST–Akt1 CA or KD (final 20 μg ml −1 ) in the presence of ATP (final 10 μM) at 30 °C for 30 min. After the phosphorylation assay, 45% of the reaction mixture was used for IP with anti-Plk1 or anti-Bad. After the wash, each immunoprecipitate was subjected to the immunoblotting. For the detection of endogenous Akt or exogenous GST–Akt1, 5% of the reaction mixture was also subjected to the immunoblotting. In vitro kinase assays using immunoprecipitated Plk1 were performed as follows. Endogenous Plk1 or exogenous Myc-Plk1 was immunoprecipitated with anti-Plk1 from HeLa cells ( Fig. 6i ) or with anti-Myc from Tet-On cells ( Supplementary Fig. S5c ), respectively. Each immunoprecipitate was washed with cell lysis buffer three times and then with reaction buffer twice. After the wash, the immunoprecipitate was incubated with or without 20 μg ml −1 of GST–Akt1 CA or KD in the reaction buffer containing 10 μM ATP at 30 °C for 30 min. After the reaction, each immunoprecipitate was subjected to immunoblotting. For the detection of endogenous Akt or exogenous GST–Akt1, 5% of cell extracts before IP and of reaction mixtures were also subjected to immunoblotting. How to cite this article: Kasahara, K. et al. PI 3-kinase-dependent phosphorylation of Plk1–Ser99 promotes association with 14-3-3γ and is required for metaphase–anaphase transition. Nat. Commun. 4:1882 doi: 10.1038/ncomms2879 (2013).